Observation of interaction-induced modulations of a quantum Hall liquid’s area Studies of electronic interferometers, based on edge-channel transport in the quantum Hall effect regime, have been stimulated by the search for evidence of abelian and non-abelian anyonic statistics of fractional charges. In particular, the electronic Fabry–Pérot interferometer has been found to be Coulomb dominated, thus masking coherent Aharonov–Bohm interference patterns: the flux trapped within the interferometer remains unchanged as the applied magnetic field is varied, barring unobservable modulations of the interference area. Here we report on conductance measurements indicative of the interferometer’s area ‘breathing’ with the variation of the magnetic field, associated with observable (a fraction of a flux quantum) variations of the trapped flux. This is the result of partial (controlled) screening of Coulomb interactions. Our results introduce a novel experimental tool for probing anyonic statistics. The behaviour of electrons and quasi-particles in mesoscopic systems stems from the combination of their wave-nature, particle-nature and the effect of Coulomb interactions. Electronic Fabry–Pérot interferometers (FPIs), and more generally ring-like geometries, have been utilized for the investigation of all these three facets [1] , [2] , [3] , [4] and the rich interplay among them [5] , [6] , [7] , [8] , [9] , [10] . In particular, electronic FPIs have possibly been the most studied candidates for probing belian and non-abelian anyonic statistics of quasi-particles in the fractional quantum Hall effect (FQHE) regime [11] , [12] , [13] , [14] . Notwithstanding considerable efforts, the experimental study of anyonic statistics is still lagging behind theory, mostly owing to the adverse effect of Coulomb interactions. Two distinct regimes in the operation of FPIs—characterized by the conductance oscillation frequencies with the applied flux—have been reported [7] , [8] and studied theoretically [15] , [16] , [17] , [18] , [19] . In the coherent AB regime, one period of these oscillations corresponds to the increase of the threaded flux through the interferometer’s area by a single flux quantum φ 0 = h / e ( e —electron charge and h —Planck’s constant) [20] . On the other hand, in the Coulomb-dominated (CD) regime, it is the mutual capacitance between the device and a modulation gate that dictates the oscillation periodicities. Interference in the AB regime is harder to observe [7] , [8] , and has not been achieved thus far in any fractional quantum Hall state. At the same time, the CD regime has its own disadvantage—it does not and cannot reveal the anyonic statistics. The AB phase underlying interference patterns evolves as 2 πδφ AB / φ 0 =2 π ( AδB + BδA 0 )/ φ 0 , where δφ AB is the variation of the threaded flux through the FPI, B the applied magnetic field, A the area enclosed by the interfering edge channel and δA 0 = α ˙ δV MG is the area variations due to the modulation gate (but excluding the effect of Coulomb interaction as explained below). Here α is the edge-channel modulation-gate mutual capacitance. The AB oscillations with δB and δV MG are hence characterized by the following frequencies: By contrast, in the CD regime with the outer most edge channel interfering, there is no B dependence of the conductance, Here, 1/ γ is the voltage required to remove a single electron from the FPI [3] , [4] , [5] , [6] , which does not depend upon the magnetic field (in similitude to the single-electron transistor [21] ). Seemingly, these two regimes may seem to be of very different nature: while the AB oscillations are due to coherent interference, the CD oscillations reflect solely the electron occupancy of the device and do not contain any information regarding the phase acquired by the interfering particles. This interpretation turned out to be too naive. A unified theoretical framework has suggested that the CD oscillations may, in fact, be AB oscillations modified by Coulomb interaction [15] . According to this interpretation [7] , [8] , [15] , as the magnetic field increases (decreases) so that the AB phase varies by AδB , the area will shrink (inflate) by δA int to keep a constant flux AδB + BδA int =0, where the subscript ‘int’ stands for ‘interactions’. This variation of the area guarantees that the charge enclosed in the interfering area is kept constant, minimizing the charging energy of the device. Then, once the flux variation reaches the value of a whole flux quantum, AδB = φ 0 , an electron abruptly ‘jumps’ from the bulk into the edge and the original area is restored [7] , [15] . According to this description, the area enclosed by the outer edge channel is ‘breathing’; on increasing the magnetic field it continuously shrinks and then abruptly inflates, altogether with periodicity Δ B = φ 0 / A . Nonetheless, the breathing in the CD regime has never been experimentally confirmed. The reason is that the measured conductance is simply constant, as the magnetic field is varied. Basically, the area response to increasing the magnetic field fully compensates the effect of the latter. The subsequent abrupt addition of an electron leads to a 2 π jump in the interference phase—clearly an unobservable effect as well. We are thus ‘blind’ to this phenomenon of area breathing. Here we report on the realization of a novel device that combines the advantages of AB interferometers with CD response. It operates in an intermediate regime—in which the area response does not fully compensate the variations of the magnetic field, rendering the area ‘breathing’ observable. In other words, , with 0< ξ <1, leading to a total phase evolution . Our main findings concerning this ‘breathing’ are summarized in equations (8, 9, 10) below. Measurements were performed on three different devices showing three distinct behaviours: AB dominated, namely, ξ =0 with no area breathing; CD, namely, ξ =1 with invisible breathing of the area; and an intermediate one ( ξ =0.75), with clear area breathing. We present conductance measurements of this novel device that incorporates both AB and CD frequencies (equations (1, 2, 3, 4)), hence contain information regarding both interference and interactions, and the interplay between them. Moreover, employing detailed analysis based on the system’s energy, we deduce the device’s charge stability diagram, providing an insight to its rich physics being ‘hidden’ in the previously reported AB and CD devices. Furthermore, we provide proposals for utilizing our device for probing anyonic statistics of quasi-particles in the FQHE regime. Experimental set-up The devices were fabricated on a GaAs-AlGaAs heterostructure, embedding a two-dimensional (2D) electron gas with electron density ∼ 2 × 10 11 cm −2 . Electron-beam and optical lithography were employed in the fabrication process, and measurements were performed at electron temperature ∼ 30 mK. All FPIs consist of a pair of quantum point contacts (QPCs), playing the role of semi-transparent mirrors ( Fig. 1 ). Three different types of devices are shown in Fig. 1 . In Fig. 1a , we show the simplest realization of a FPI; such FPIs have high charging energy, regardless of their size [7] , [8] , [22] , thus showing CD behaviour. Tto suppress Coulomb interactions, a small Ohmic contact (106 nm Au/53 nm Ge/40 nm Ni with surface area 0.5 μm 2 alloyed to the heterostructure) is placed at the centre of the interferometer’s bulk [22] ( Fig. 1b , gold, false colour; see Methods for more information regarding the Ohmic contact). Such devices show AB behaviour [22] . A third type of device, not reported previously (to the best of our knowledge), consists of placing such Ohmic contacts in the vicinity of the FPI, as depicted in Fig. 1c . Unexpectedly, we have found that in such a device, the suppression of the Coulomb interactions is less efficient than the centre Ohmic contact, yet it is still significant, giving rise to a new regime intermediate between AB and CD. The role of this Ohmic contact placed in the device’s vicinity is to screen the Coulomb interactions via its capacitance to the interferometer’s bulk (increasing C bulk while maintain C eb intact, see definitions in Discussion below and more details in Methods), effectively lowering the device’s charging energy and decreasing the interaction parameter ξ . All three devices were fabricated on the same heterostructure and designed to have the same size A ≈2.5 μm 2 so that they differ merely by the presence and the position of the Ohmic contacts. A fourth type of device, with the Ohmic contact inside its bulk, and surrounded by an additional gate was found to operate in the intermediate regime as well, and is discussed in Supplementary Note 1 and Supplementary Figs 1–3 . All measurements were conducted at bulk fillings 1< ν B <2, with the outer most edge-channel interfering. 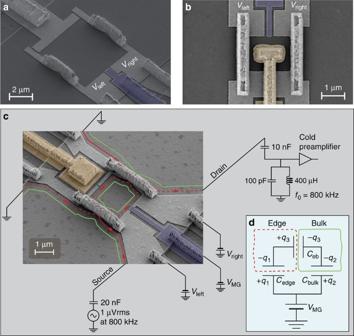Figure 1: Scanning electron microscopy images and an illustration of the experimental set-up. (a) Bare FPI; such devices show distinct Coulomb dominated (CD) behaviour. (b) FPI with a grounded Ohmic contact in its centre (gold, false colour) aimed at screening Coulomb interactions; such devices show Aharonov–Bohm (AB) interference. (c) FPI with a grounded Ohmic contact in its close proximity (gold, false colour), inducing partial screening of Coulomb interactions; such devices show intermediate behaviour between the CD and AB. Red lines represent edge states and arrows represent the current’s chirality. Current is injected into the device from the source, partitioned at the two QPCs, and probed at the drain employing a cold amplifier. Partitioned current is denoted by dashed lines. Modulation gates are marked by blue (false colour) in all images. (d) An equivalent electric circuit model describing the interferometer system with filling factor 1<vB<2. The system consists of the lowest Landau level’s edge (denoted as ‘edge’), the bulk (denoted as ‘bulk’) and the modulation gate. The mutual capacitances between all three,Ceb,CedgeandCbulk, are marked on top of the circuit. The excess charge on the edge is denotedδQedge=δq3−δq1, while the excess charge in the bulk is. Further details on the capacitive model are provided in analysis, as well as inSupplementary Note 2andSupplementary Fig. 5. Figure 1: Scanning electron microscopy images and an illustration of the experimental set-up. ( a ) Bare FPI; such devices show distinct Coulomb dominated (CD) behaviour. ( b ) FPI with a grounded Ohmic contact in its centre (gold, false colour) aimed at screening Coulomb interactions; such devices show Aharonov–Bohm (AB) interference. ( c ) FPI with a grounded Ohmic contact in its close proximity (gold, false colour), inducing partial screening of Coulomb interactions; such devices show intermediate behaviour between the CD and AB. Red lines represent edge states and arrows represent the current’s chirality. Current is injected into the device from the source, partitioned at the two QPCs, and probed at the drain employing a cold amplifier. Partitioned current is denoted by dashed lines. Modulation gates are marked by blue (false colour) in all images. ( d ) An equivalent electric circuit model describing the interferometer system with filling factor 1< v B <2. The system consists of the lowest Landau level’s edge (denoted as ‘edge’), the bulk (denoted as ‘bulk’) and the modulation gate. The mutual capacitances between all three, C eb , C edge and C bulk , are marked on top of the circuit. The excess charge on the edge is denoted δQ edge = δq 3 − δq 1 , while the excess charge in the bulk is . Further details on the capacitive model are provided in analysis, as well as in Supplementary Note 2 and Supplementary Fig. 5 . Full size image Observations Tuning the magnetic field to the ν B =2 plateau and partitioning the outer edge channel, conductance oscillations are measured as function of δB and δV MG , with the different FPIs shown in Fig. 1 . For the device shown in Fig. 1b , constant-phase lines in the B - V MG 2D plane follow a negative slope—a typical result in the AB regime ( Fig. 2a ). A fast Fourier transform (FFT) extracts —agreeing well with the lithographically enclosed area, and —needed to remove one flux quantum from the interior of the device (equations (1 and 2)). For the device shown in Fig. 1a , no oscillation as function of δB is observed—in agreement with the prediction for the CD regime (equations (3 and 4))—with a modulation-gate frequency —needed to remove one electron. 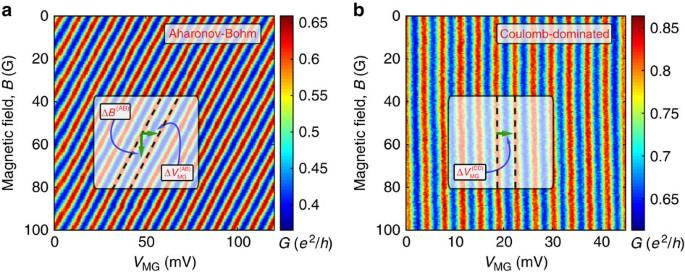Figure 2: Conductance versus modulation-gate voltageδVMGand magnetic fieldδB measured with Aharonov Bohm dominated and Coulomb-dominated devices. (a) 2D conductance measured with the FPI with an Ohmic contact in its centre (seen inFig. 1b) atB=4.7 T. This plot shows a clear AB behaviour: constant-phase lines are marked with grey lines and the AB periodsand ΔB(AB)are marked accordingly. (b) 2D conductance measured with the bare FPI (seen inFig. 1a) atB=4.7 T. This plot shows a clear CD behaviour with no dependence of the conductance on magnetic field; constant-phase lines are marked with grey lines and the CD periodis marked accordingly. Figure 2: Conductance versus modulation-gate voltage δV MG and magnetic field δ B measured with Aharonov Bohm dominated and Coulomb-dominated devices. ( a ) 2D conductance measured with the FPI with an Ohmic contact in its centre (seen in Fig. 1b ) at B =4.7 T. This plot shows a clear AB behaviour: constant-phase lines are marked with grey lines and the AB periods and Δ B (AB) are marked accordingly. ( b ) 2D conductance measured with the bare FPI (seen in Fig. 1a ) at B =4.7 T. This plot shows a clear CD behaviour with no dependence of the conductance on magnetic field; constant-phase lines are marked with grey lines and the CD period is marked accordingly. Full size image Turning to employing the device in Fig. 1c , we commenced by measuring the conductance for rather pinched QPCs (< t >=0.05), shown in Fig. 3a . This lattice-like conductance plot represents the charge stability diagram of the device and contains information both on the interference and on the device’s charging, as we elaborate in Discussion. Although this plot is rather complex, its 2D FFT, shown in Fig. 3b , is simple; it reveals a lattice of peaks (as expected from an FFT of a lattice) all being linear combinations of underlying AB and CD frequencies, denoted on top of the figure. We find and for the AB frequencies, and 1/Δ B (CD) =0 and for the CD frequencies. These frequencies are found relatively close to the ones of the ‘pure AB’ and ‘pure CD’ cases extracted from Fig. 2a,b , respectively. Furthermore, we find to be the only frequency that depends on magnetic field (in the tesla range), as anticipated from equations (1, 2, 3, 4) ( Supplementary Fig. 4 ). 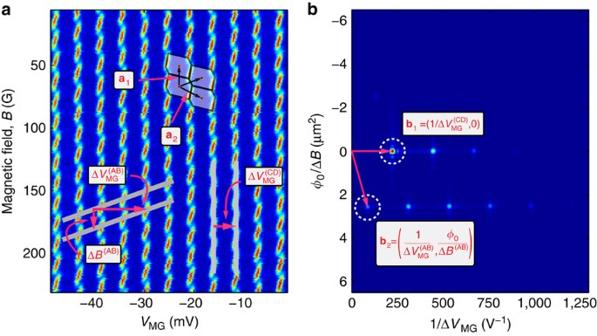Figure 3: Conductance of a FPI operating in an intermediate regime as a function of the modulation-gate voltageδVMGand the magnetic fieldδB. (a) 2D conductance measured with the FPI with an Ohmic contact in its vicinity (seen inFig. 1c) atB=5 T, giving rise to a charge stability diagram. The vectors marked on top of the figure connect different cell and can be translated to physical processes, as elaborated in analysis. Grey lines mark the underlying AB and CD frequencies. (b) 2D FFT of the conductance ina, revealing a clear lattice structure as well, as expected from an FFT of a lattice. The underlying AB and CD frequencies, marked by two vectors (b1andb2. respectively, highlighted with white dashed circles), span this Fourier lattice, and the reason for their appearance here is elaborated in analysis. Figure 3: Conductance of a FPI operating in an intermediate regime as a function of the modulation-gate voltage δV MG and the magnetic field δ B. ( a ) 2D conductance measured with the FPI with an Ohmic contact in its vicinity (seen in Fig. 1c ) at B =5 T, giving rise to a charge stability diagram. The vectors marked on top of the figure connect different cell and can be translated to physical processes, as elaborated in analysis. Grey lines mark the underlying AB and CD frequencies. ( b ) 2D FFT of the conductance in a , revealing a clear lattice structure as well, as expected from an FFT of a lattice. The underlying AB and CD frequencies, marked by two vectors ( b 1 and b 2 . respectively, highlighted with white dashed circles), span this Fourier lattice, and the reason for their appearance here is elaborated in analysis. Full size image Moreover, by further opening the confining QPCs to < t >=0.7, the presence of abrupt jumps in the conductance (phase jumps) becomes more clear ( Fig. 4a ), which shows good agreement with the conductance’s model that stems from the minimization of the system’s energy ( Fig. 4b ; see Discussion below; Supplementary Notes 2–3 ; Supplementary Fig. 5–9 ). 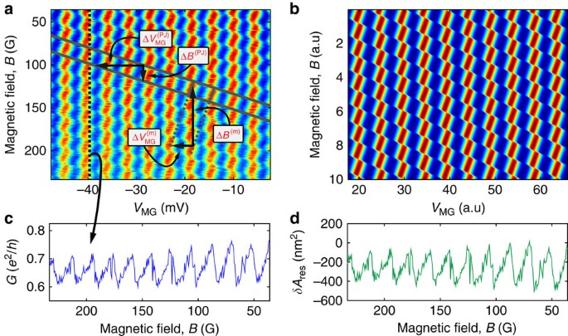Figure 4: 2D conductance plot with clear phase jump lines. (a) Conductance is measured with the same device asFig. 3, but with substantially higher transmission (<t>≈0.7). Phase jump lines are marked by solid descending lines and the frequency defined by their slope is marked byand ΔB(PJ). In between adjacent phase jump lines, we have continuous conductance oscillations. By extrapolating these continuous oscillations (dashed ascending lines), we may attribute them periodicities denotedand ΔB(m). More details are provided in analysis. (b) Theoretical plot, simulated according to the conductanceGexpressed in Discussion. (c) ConstantδVMGline taken froma, showing clear phase accumulation followed by abrupt phase jump of, which is also equal to the value ofξ(equation (11)). (d) The area responseδAintinferred from the conductance’ phase (c). The relation between the area response and the phase is obtained by inverting the relation betweenδAintand the conductanceG, provided in the caption ofFig. 5. Note that indeed (c,d) are highly similar (as anticipated by the theoretical plots, cf. yellow curves inFig. 5d,b), but they are not identical. Naturally, for small values of the phase, the conductance is nearly proportional to it. Figure 4: 2D conductance plot with clear phase jump lines. ( a ) Conductance is measured with the same device as Fig. 3 , but with substantially higher transmission (< t >≈0.7). Phase jump lines are marked by solid descending lines and the frequency defined by their slope is marked by and Δ B (PJ) . In between adjacent phase jump lines, we have continuous conductance oscillations. By extrapolating these continuous oscillations (dashed ascending lines), we may attribute them periodicities denoted and Δ B (m) . More details are provided in analysis. ( b ) Theoretical plot, simulated according to the conductance G expressed in Discussion. ( c ) Constant δV MG line taken from a , showing clear phase accumulation followed by abrupt phase jump of , which is also equal to the value of ξ (equation (11)). ( d ) The area response δA int inferred from the conductance’ phase ( c ). The relation between the area response and the phase is obtained by inverting the relation between δA int and the conductance G , provided in the caption of Fig. 5 . Note that indeed ( c , d ) are highly similar (as anticipated by the theoretical plots, cf. yellow curves in Fig. 5d,b ), but they are not identical. Naturally, for small values of the phase, the conductance is nearly proportional to it. Full size image Analysis Since the AB and CD types of behaviour are merely two different regimes of operation of the same device, they may be analysed within the same theoretical framework [15] . We address a set-up, where transport through the outer most edge channel at 1< ν B <2 gives rise to interference. This case has been studied experimentally. We denote the charge added to the lowest Landau level (lowest LL) by Q ↓ , and that added to the upper Landau level (upper LL) by δQ ↑ . Hereafter, we refer to the interfering outer most edge channel (compressible ring belonging to the lowest LL) as the ‘edge’, and to the rest of the charge inside the FPI as ‘bulk’ [23] . The charge variations in the edge and bulk are denoted δQ edge and δQ bulk , respectively. We note that for any device without an Ohmic contact within its centre, δQ ↑ changes discretely accounting for the localized charges in the bulk [15] , [16] . We consider a minimal capacitive model for describing the FPI set-up [15] , [16] , [24] depicted in Fig. 1d . The model consists of three capacitances C edge , C bulk and C eb describing the mutual Coulomb interactions between the system’s three components, δQ edge , δQ bulk and δV MG . The total energy of the system can then be written as the sum of three contributions [15] , [17] , [25] , [26] , E total = E eb + E edge + E bulk , where the second and third terms are the edge and bulk charging energies (depending solely on δQ edge and δQ bulk , respectively), and the first term is due to the interaction between them. This first term can be presented as function of their sum δQ edge + δQ bulk . The relation between this approach and an earlier one (cf. ref. 15 ), where the variable δQ edge · δQ bulk have been employed, is discussed in Supplementary Note 2 . The system’s charge state is determined by minimizing the total energy E total . In the quantum Hall regime, the charge added to the lowest LL, δQ ↓ , follows the total flux, δφ tot , enclosed by the latter: as the flux increases (decreases), single-particle states cross in below (cross in above) the Fermi energy, increasing (decreasing) the number of occupied states: Here, in the third term on the right hand side, δA int represents the interaction-induced area response. Thus, the overall variation of the area δA = δA 0 + δA int is separated into two components. The first component is a linear component that is solely a result of variations of the modulation-gate voltage, δA 0 = αBδV MG , and stems solely from its mutual capacitance to the interfering edge. The second component is an oscillating component [7] , [15] , δA int , which is a function of both δB and δV MG , for which we derive the full expression below (and allowing us to present the total phase as an explicit function of δB and δV MG , cf. equation (8) below). Magnetic field variations As the magnetic field increases and the filling factor decreases, charge is removed from the upper Landau level into the lowest Landau level. More precisely, with every flux quantum added, the degeneracy each Landau level increases by one; resulting in a transfer of a single electron from the upper LL (hence δQ ↑ =±1) to the lowest LL (hence δQ ↓ =±1), while keeping the total charge in the system constant. The corresponding variation of energy can be expressed in terms of δQ ↑ and δQ ↓ [15] , [27] : where δQ tot = δQ ↓ + δQ ↑ , , and all three coefficients are related to the relevant different capacitances [15] : are system specific, with D =( C edge + C eb )( C bulk + C eb )− . Equation (6) implies that the energy is minimized if and , leading to δQ tot =0 at all times. This continuous charging of the edge, δQ ↓ , should result in the periodicity Δ B = φ 0 / A . The latter coincides with the behaviour in the AB regime, as seen in Fig. 2a , measured with the device shown in Fig. 1b . In this device, while δQ ↓ is continuously charged from the leads, δQ ↑ is discharged into the centre Ohmic contact. Previous measurements have also reported the observations of AB oscillations even without the centre Ohmic contact, but rather with a top gate covering the device [7] , [8] . In that case, the upper LL’s charge δQ ↑ cannot vary continuously (as in the case with an Ohmic contact at the centre of the device), but rather discretely, because the upper LL is isolated by an incompressible strip [15] , [23] . Thus, as the magnetic field increases such that AδB < φ 0 , the lowest LL is continuously charged by , leading to an increase of the total charge with δQ ↑ =0 due to the upper LL’s charge quantization. This of course will increase the charging energy (which favors δQ tot =0; first term in equation (6)), which is possible since the top gate effectively decreases K EB (and thus C eb ), such that K EB << K E (and C eb << C bulk ) [7] , [8] , [15] . Then, once a whole flux quantum is added AδB = φ 0 , the energy can again be minimized by discharging the upper LL abruptly δQ ↑ =− e . This AB behaviour is summarized in Fig. 5a–c (blue), leading to a conductance depicted in Fig. 5d (blue). 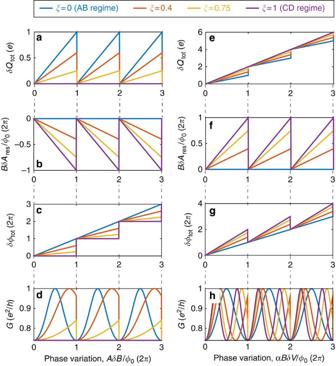Figure 5: Theoretical plots for the Fabry–Pérot interferometer in all regimes. (a) Total charge in the system,δQtot=δQ↓+δQ↑. (b) The area responseδAint. (c) The total fluxδφtot, including both the externally varied phaseAδB/φ0and the responseBδAint/φ0. (d) The resulting conductance for relatively open QPCs (t2=0.85), taking the straightforward form(further details are provided inSupplementary Note 3). All four graphs (a–d) are plotted versus variations of the magnetic field. (e–h) Similar graphs asa–d, as a function of modulation-gate voltageδVMG. The plots are given for the simple case ofνB=2. For simplicity, we plote–hin the caseCbulk=Cedgeat bulk filling factorνB=2, leading to a CD frequency that is twice of the AB frequency. The choice of these values does not change the qualitative picture, and we note that we findCbulk=1.45˙Cedgein the experiment, deduced from the measured frequencies. Figure 5: Theoretical plots for the Fabry–Pérot interferometer in all regimes. ( a ) Total charge in the system, δQ tot = δQ ↓ + δQ ↑ . ( b ) The area response δA int . ( c ) The total flux δφ tot , including both the externally varied phase AδB / φ 0 and the response BδA int / φ 0 . ( d ) The resulting conductance for relatively open QPCs ( t 2 =0.85), taking the straightforward form (further details are provided in Supplementary Note 3 ). All four graphs ( a – d ) are plotted versus variations of the magnetic field. ( e – h ) Similar graphs as a – d , as a function of modulation-gate voltage δV MG . The plots are given for the simple case of ν B =2. For simplicity, we plot e – h in the case C bulk = C edge at bulk filling factor ν B =2, leading to a CD frequency that is twice of the AB frequency. The choice of these values does not change the qualitative picture, and we note that we find C bulk =1.45˙ C edge in the experiment, deduced from the measured frequencies. Full size image On the other hand, as alluded above in the CD regime, the total charge must be constant at all times due to the large charging energy K EB ≫ K E , thus C eb ≫ C bulk (in the absence of an Ohmic contact or top gate). As a result, when the applied magnetic field is increased, the area shrinks to prevent the enclosed flux from increasing. This means , with δQ ↓ =0 due to the bulk’s quantization, leading to δA int =− AδB / B . In that case, as the interferometer’s area shrinks, a dipole is created: a depleted region (positively charged) is created just outside the boundary of the shrinking interferometer, while an excess negative charge accumulates inside. The energy increase due to this dipole is reflected by the second and third terms in equation (6). Once a whole flux quantum is added AδB = φ 0 , the energy can again be minimized by abruptly moving an electron from the upper LL to the lowest LL, described by the simultaneous variation δQ ↑ =− e and δQ ↓ =+ e . At this point, the area response δA int should abruptly vanish from ∼ 810 nm 2 (a flux quantum’s area at 5 T) to 0 μm 2 . Such an abrupt response cannot be inferred from the measured conductance ( Fig. 2b ), since it should result in a 2 π variation of the Aharonov–Bohm phase. This leaves the conductance constant as function of δB . This CD behaviour is summarized in Fig. 5a–c (purple), leading to a conductance depicted in Fig. 5d (purple). To summarize, for any device without an Ohmic contact within its centre (implying a quantization condition on δQ ↑ ), the system ‘decides’ whether it shrinks or not, and by how much, according to the values of K EB and K E . Taking the derivative of the total energy with respect to δA int , we obtain δA int =− ξ · AδB / B , with . The AB regime corresponds to the limit K E ≫ K EB , leading to ξ =0 and δA int =0; the CD corresponds to the limit K E << K EB , leading to ξ =1 and δA int =− AδB / B . The behaviour in the intermediate regime is summarized in Fig. 5a–c (red and yellow for ξ =0.25 and ξ =0.75, respectively), resulting in the conductance depicted in Fig. 5d . The theoretical prediction ( ξ =0.75; Fig. 5d , yellow) is consistent with the measured conductance shown in Fig. 4c , from which we have retrieved both the area=2.6 μm 2 (from the main periodicity) and the interaction parameter ξ =0.75 (from the amplitude of the phase jumps). The possibility to extract these two parameters from a single magnetic field scan demonstrates the versatile information contained in the intermediate regime—it incorporates both interactions (quantified by ξ ) and interference (related to A ). Furthermore, from the conductance ( Fig. 4c ), we infer the evolution of the area response, δA int , as function of δB , shown in Fig. 4d . We find a maximal area response of δA int =500 nm 2 , which is in good agreement with our expectation . Modulation-gate variations The two handles we have, varying the magnetic field δB and varying the modulation-gate voltage δV MG , are substantially different from each other. While in both AB and CD regimes, the total charge must be conserved for δB variations on the scale of several flux quanta, AδB ≫ φ 0 , δV MG induces charge on the device through its capacitance γ : applying δV MG requires charging the device by δQ tot = γδV MG that divides into each Landau levels [15] , [16] : and . Thus, the energy variation of the system (equation (6)) can be reformulated as: Although equation (7) is valid for any variation of δB and δV MG , only modulation-gate variations, δV MG , are considered in this section. In the AB regime, as the modulation-gate voltage increases by δV MG such that , the lowest LL is continuously charged by allowing us to observe Aharonov–Bohm interference with a period (cf. Fig. 2a ). Note that α is independent to the magnetic field ( Supplementary Fig. 4 ). Simultaneously, we expect the upper LL to be continuously charged from the centre Ohmic contact, satisfying . Alternatively, with top-gated devices ( K EB << K E ), the upper LL acquires an additional electron discretely only once this last expression (which can be regarded as the induced charge in the bulk) amounts to an increase by a whole-electron charge . This AB behaviour is summarized in Fig. 5e–g (blue) and results in a conductance depicted in Fig. 5h (blue). By contrast, in the CD regime, the high charging energy K EB << K E requires for all values of δV MG . As δQ ↑ =0 due to charge quantization in the upper LL, it follows that . According to equation (5), this necessitates an area response , (which is always larger than zero since ; see Supplementary Figs 2 and 4 ). Namely, while in the AB regime the area dilations are dictated solely by the mutual capacitance between the edge and the modulation gate, α , here, in the CD regime, the area dilations overshoots to satisfy the capacitance of the device (including both the edge and the bulk) to the modulation gate, γ . This overshoot will cost an energy proportional to K E (equation (7)). Then again, once this overshoot is equivalent to a whole electron, the area will retract back minimizing the total energy. This CD behaviour is summarized in Fig. 5e–g (purple) and results in a conductance depicted in Fig. 5h (purple). Similarly to the analysis of magnetic field variations, we can express the area response to variations of δV MG for any value of the interaction parameter ξ : we obtain resulting in a total area variation . This is summarized in Fig. 5e–h (red and yellow for ξ =0.25 and ξ =0.75, respectively). Analysis of the entire B − V MG plane So far, we have analysed the area response to variations of either δB or δV MG . We now turn our attention to concomitant variations of both. This will allow us to analyse the data shown in Figs 3a and 4a . Notably, the interference pattern in Figs 3a and 4a may be decomposed into two ingredients. First, descending lines along which phase jumps take place (cf. solid lines in Fig. 4a ). The respective periodicities are denoted and Δ B (PJ) (marked on top of Fig. 4a , with the superscript ‘PJ’ for ‘phase jump’). Second, continuous conductance oscillations with respect to modulation-gate voltage and magnetic field in between two adjacent phase jump lines. The corresponding periodicities are then and Δ B (m) ,respectively (marked on top of Fig. 4a as well, with the superscript ‘m’ for ‘modified’). These continuous oscillations reflect the interference of electrons at the edge. Crossing a maximal conductance line (for example, following arrow a 2 in Fig. 3a ) corresponds to an incremental variation of δQ ↓ by ± e . Here, ‘modified’ alludes to the fact that these continuous oscillations are in fact coherent AB oscillations modified by the Coulomb interaction. Likewise, crossing a phase jump line (for example, following arrow a 1 in Fig. 3a ) implies a change of the upper LL’s charge δQ ↑ by ± e . Naturally, the combination of these two types of processes gives rise to the system’s charge stability diagram in the B − V MG plane. To express the modified periodicities Δ B (m) and (in between abrupt changes of the charge), we need to determine an expression for the interference phase (equation (5)) for a fixed number of electrons in the upper LL. We first generalize the dependence of the area response on δB and δV MG by combining the results obtained in the previous sections: , where the last term represents phase jumps that accompany variations of δQ ↑ =± e (for further details see Supplementary Notes 2–3 ). This result is then plugged into the expression for the total phase (equation (5)) [15] : Note that the last term of the of the equation accounts for abrupt phase jumps. The respective modified periodicities are: These two frequencies are notably a linear combination of the AB and CD frequencies (cf. equations (1, 2, 3, 4)): and . Constant flux lines of δφ tot follow a negative slope in the B − V MG plane, similar to the pure AB case. We extract Δ B (m) =65.9 G and from our data; each of these periodicities leads to an interaction parameter ξ =0.75±0.01. The periodicities associated with phase jumps are found to be and (cf. equations (1, 2, 3, 4); see Supplementary Note 3 for details). We find this relation to be in agreement with the measured values. Note that these periodicities do not depend on the value of ξ . Combining the modified periodicities (equations (9 and 10)) with the phase jump periodicities allows us to construct the charge stability diagram. Naturally, vectors connecting different cells in the diagram ( Fig. 3a ) represent different discrete charge variations ( δQ ↓ , δQ ↑ )=( n , m ) (cf. Supplementary Note 2 ). It is convenient to select the following basis ( Fig. 3a ): and . Here, a 1 represents the process of moving one electron from the upper to the lowest LL (namely, n =1 and m =−1, as explained in ‘magnetic field variations’), while a 2 represents adding one electron to the lowest LL and keeping the upper LL’s charge constant (namely, n =1 and m =0). Evidently, their sum a 1 + a 2 refers to adding one electron to the upper LL, while keeping the lowest LL’s charge constant. The reciprocal lattice is spanned by the pure AB and CD frequencies, and respectively (cf. Fig. 3b ). Phase jumps and proposed experiments Finally, we study qualitatively the phase jump taking place when a phase jump line is crossed, following an infinitesimal variation of either δB or δV MG . The acquired phase is given by [15] : Evidently, in the extreme AB and CD cases this phase jump is zero ( ξ =0) or unobservable ( ξ =1), respectively. Experimentally, the value of ξ (0< ξ <1) can be deduced from directly measuring the phase jump (seen in Fig. 4c ). We find ξ ≈0.75 (similar to the value we obtained independently by comparing the measured frequencies with equations (9 and 10) of the previous section). This value of ξ corresponds to an area jump of 440 nm 2 (cf. Fig. 4d ). A possible extension of our analysis to the FQHE regime is straightforward and results in a phase jump given by: where θ stat is the quasi-particles’ statistical braiding phase (for example, for anyons at ν B =1/3). While the difference between equation (11) and equation (12) is seemingly minute, its impact might be significant. It is apparent that, by probing Δ θ in a fractional filling factor, the requirement for probing θ stat is 0≤ ξ <1. This requirement is to be compared with previous measurements that focused on a pure AB, ξ =0 and pure CD, ξ =1 (anyonic statistics cannot be probed). Breaking this dichotomy between the pure AB and pure CD regimes thus provides us with a toolbox to probe anyonic statistics. We stress that the protocol to probe fractional statistics requires the study of the conductance as function of the magnetic field and the modulation-gate voltage (similarly to Figs 3a and 4a ). This is needed to identify the regime of operation (the parameter ξ ) with no ambiguity. Previous reports [28] , [29] presenting conductance oscillations in fractional filling factors have failed to show such 2D scans of the conductance in a 2D parameter space, and were thus criticized for not excluding a CD behaviour, or for being otherwise inconclusive [8] , [19] , [30] . Other works, which did identify the regime of operation, simply failed to obtain an AB behaviour in fractional filling factors. These attempts utilized both large area and small area devices. For the former, Coulomb effects are expected to be negligible if a top gate is placed on top of the sample [7] , [8] or an Ohmic contact is placed at the centre of the device [22] , rendering the regime of operation AB. Yet an AB interference pattern (observable in the integer quantum Hall effect regime) has not been observed for fractional filling factors. This might be attributed to a short coherence length of anyons in such relatively large devices. One may then resort to smaller FPIs. Unfortunately, reducing the device’s size leads to the undesired CD regime in the case of top-gated devices [7] , [8] , and, in the case of devices with Ohmic contacts at the centre, further miniaturization is limited. The device reported here, having an Ohmic contact placed outside its circumference, operates in a regime intermediate between AB and CD. Given the possibility to make the device’s size small in such a design, yet maintaining ξ <1 with a clear signature of coherent Aharonov–Bohm oscillations, presents us with an intriguing prospects: notwithstanding a short quasi-particle coherence length, coherency may still be maintained over the size of the interferometer. Interference signal, a smoking gun evidence for anyonic statistics, is then potentially observable. We provide here an experimental evidence of area modulations of a FPI implemented in the quantum Hall effect regime. These modulations stem from the minimization of the system’s energy, as the applied magnetic field and the modulation-gate voltage are varied. Our analysis does not rely on the coherent operation of the device. The measurement of the area modulations, though, could be realized through the observation of coherent interference oscillations. The area evolution consists of a continuous shrinking when increasing magnetic field, followed by an abrupt dilation. We have employed a theoretical framework that accounts for both the AB and the CD, and a novel intermediate regime. The latter enables us to construct the system’s charge stability diagram as well, showing good agreement with a minimal theoretical model. Both the area breathing and the charge stability diagram are used towards a complete characterization of the device, the latter being hidden in the pure AB or CD limits. Utilizing a similar interferometer operating in the intermediate regime in the domain of the FQHE regime is called for. The novelty of our device lies within the possibility to explore a wide range of the interaction parameter ξ , in which the quasi-particles’ braiding statistics is observable. In other words, our findings reported here pave a new path for probing anyonic statistics in the FQHE regime. Ohmic contacts As explained in the text, the ‘pure’ CD regime can be avoided through undermining the effect of Coulomb interactions. This can be achieved utilizing two different methods: First: we place a grounded Ohmic contact inside the interferometer’s bulk, thus avoiding its charge quantization (cf. the device in Fig. 1b ). The Ohmic contact consists of 106 nm Au/53 nm Ge/40 nm Ni alloyed to the heterostructure having a resistance of 500 Ω at zero magnetic field. This Ohmic contact is not resistively coupled to the edge (the observed coherent phase oscillations are evidence to that). This important point has been verified in a previous work (cf. Supplementary Fig. 9 in ref. 22 ), employing a more complex set-up. The latter consisted of a FPI with a centre contact and an additional QPC placed along the interferometer’s edge, allowing to reflect edge channels selectively into the centre Ohmic contact. Then, by measuring the current at the centre contact, we have verified that it is non-vanishing only once the chiral channel corresponding to the LLL is physically reflected into this contact. Second: this consists of lowering the device’s charging energy, K EB . For this purpose, two schemes are available. One scheme consists of covering the whole area of the FPI by a metallic top gate, increasing its capacitance, thus lowering its charging energy [7] , [8] . This scheme has not been utilized in our measurements, but has been reported to work well for relatively large FPIs (areas >12 μm 2 ) [7] , [8] , resulting in a ‘pure’ AB behaviour. On the other hand, devices of area <4 μm 2 have been found to operate in the CD regime, even if covered by top gate [7] , [8] . This was attributed to the different scaling of the capacitances C eb and C bulk with area [15] . The other scheme relies on placing an Ohmic contact in the vicinity of the interferometer. The role of the Ohmic contact here can be understood through a mutual capacitance C ob between the Ohmic contact and the bulk, similar to the effect of top gates [7] , [8] ; we find, though, that this placement of an Ohmic contact is substantially more effective than a top gate. The mutual capacitance effectively increases the capacitance of the bulk ( C bulk → C bulk + C ob ), accounting for the partial screening by the Ohmic contact, while keeping the capacitance between the edge and the bulk unchanged ( C eb → C eb ). This leads to a decrease of the interaction parameter, ξ ( ξ =0.75 in the results reported here, compared with ξ =1 with top-gated devices of the same size 4 μm 2 ). As is discussed in the main text, this new design gives rise to the intermediate regime. Measurement techniques Our electronic set-up for conductance measurements is depicted in the Fig. 1c . We note that two amplifiers were used in the course of our measurements; the first, a homemade voltage preamplifier at T =1 K having a gain factor ∼ 10 and a commercial amplifier (NF SA-220F5) at room temperature having a voltage gain ∼ 200. All experiments are performed within 3 He– 4 He dilution fridges. Electron temperatures are measured via shot-noise measurements by driving a variable d.c. source current at a centre frequency of 800 kHz and bandwidth of 10 kHz. Data availability The data that support the findings of this study are available from the corresponding author upon request. How to cite this article: Sivan, I. et al. Observation of interaction-induced modulations of a quantum hall liquid’s area. Nat. Commun. 7:12184 doi: 10.1038/ncomms12184 (2016).